Uncoupling of the endocannabinoid signalling complex in a mouse model of fragile X syndrome Fragile X syndrome, the most commonly known genetic cause of autism, is due to loss of the fragile X mental retardation protein, which regulates signal transduction at metabotropic glutamate receptor-5 in the brain. Fragile X mental retardation protein deletion in mice enhances metabotropic glutamate receptor-5-dependent long-term depression in the hippocampus and cerebellum. Here we show that a distinct type of metabotropic glutamate receptor-5-dependent long-term depression at excitatory synapses of the ventral striatum and prefrontal cortex, which is mediated by the endocannabinoid 2-arachidonoyl- sn -glycerol, is absent in fragile X mental retardation protein-null mice. In these mutants, the macromolecular complex that links metabotropic glutamate receptor-5 to the 2-arachidonoyl- sn -glycerol-producing enzyme, diacylglycerol lipase-α (endocannabinoid signalosome), is disrupted and metabotropic glutamate receptor-5-dependent 2-arachidonoyl- sn -glycerol formation is compromised. These changes are accompanied by impaired endocannabinoid-dependent long-term depression. Pharmacological enhancement of 2-arachidonoyl- sn -glycerol signalling normalizes this synaptic defect and corrects behavioural abnormalities in fragile X mental retardation protein-deficient mice. The results identify the endocannabinoid signalosome as a molecular substrate for fragile X syndrome, which might be targeted by therapy. Fragile X syndrome (FRAX), the most frequently known genetic cause of autism, is characterized by a series of physical, cognitive and emotional symptoms that include social deficits and diminished ability to learn [1] . FRAX is due to the mutation of a single gene, called FMR1 (ref. 2 ), which encodes for the fragile X mental retardation protein (FMRP) [3] . FMRP regulates the translation and transport of messenger RNAs in dendritic spines of brain neurons, and is involved in modulating signal transduction through type-I metabotropic glutamate (mGlu 1 and mGlu 5 ) receptors at glutamatergic synapses throughout the brain. Loss of FMRP causes profound changes in the structure of neuronal dendrites and enhances, in the hippocampus and cerebellum of FMRP-deficient ( fmr1 −/− ) mice, a form of long-term depression (LTD) that requires mGlu 5 receptor-mediated protein synthesis [3] , [4] , [5] , [6] , [7] . In medium spiny neurons of the ventral striatum and pyramidal neurons of the prefrontal cortex (PFC), activation of mGlu 5 receptors initiates a distinct form of LTD, which does not depend on protein synthesis and is affected by the retrograde endocannabinoid (eCB) transmitter, 2-arachidonoyl- sn -glycerol (2-AG) [8] , [9] . Stimulation of mGlu 5 receptors releases 2-AG through the sequential recruitment of two enzymes: phospholipase C-β, which produces 1,2-diacyl- sn -glycerol, and diacylglycerol lipase-α (DGL-α), which converts 1,2-diacyl- sn -glycerol into 2-AG [10] , [11] , [12] . Morphological studies have shown that both phospholipase C-β and DGL-α are localized to the perisynapse, a subdivision of the dendritic spine that forms a 100–200-nm-thick border around the postsynaptic density [13] . mGlu 5 receptors are concentrated in this region [14] where they may be physically linked to DGL-α through the adaptor protein Homer [10] , [15] . This supramolecular complex is likely to have an important role in eCB-mediated transmission at excitatory synapses, by providing a focal point for the generation of a 2-AG pool that is specifically committed to retrograde transmission. The 2-AG produced by this complex can readily cross the synaptic cleft to access CB 1 cannabinoid receptors on presynaptic terminals, where the 2-AG-deactivating enzyme monoacylglycerol lipase (MGL) is also found [16] , [17] . We propose that this complex, which we refer to as 'eCB signalosome', allows for the separation of the 2-AG pool responsible for eCB signalling from other cellular pools of 2-AG, such as those involved in eicosanoid production and phospholipid remodelling. FMRP deletion is known to be associated with greater eCB-mediated responses at GABAergic synapses of the dorsal striatum and CA1 region of the hippocampus [18] , [19] . Here, we show that loss of FMRP is accompanied by marked deficits in mGlu 5 -dependent 2-AG release and eCB-mediated LTD at excitatory synapses of the forebrain, as well as by a structural disorganization in the eCB signalosome. We further show that inhibition of presynaptic MGL activity normalizes eCB-mediated LTD and corrects key behavioural abnormalities in fmr1 −/− mice, suggesting that pharmacological enhancement of 2-AG signalling might offer a new therapeutic strategy for FRAX. FMRP binds DGL-α mRNA and controls 2-AG signalling FMRP regulates protein translation in postsynaptic spines by interacting with mRNAs that often, albeit not always, contain a G-quartet FMRP-binding motif [20] . A bioinformatics search showed that an FMRP-binding sequence is present in DGL-α mRNA ( Fig. 1a ), but not in mRNAs encoding for structurally or functionally related enzymes such as DGL-β, MGL, N -acylphosphatidylethanolamine-selective phospholipase D (NAPE-PLD) and α/β hydrolase domain-6 (ABHD6) (data not shown). To test whether FMRP binds the DGL-α message, we immunoprecipitated FMRP from mouse forebrain homogenates and used quantitative PCR to measure DGL-α mRNA in the pellets. The pellets contained DGL-α mRNA ( Fig. 1b ), but no detectable levels of mRNAs encoding for DGL-β or NAPE-PLD ( Fig. 1c ). As expected, the precipitates also contained mRNAs encoding for PSD-95 and amyloid precursor protein, which are known to bind FMRP [21] , [22] ( Fig. 1d ). Moreover, experiments with rat cortical neurons in primary cultures showed that exposure to the mixed mGlu 1 /mGlu 5 receptor agonist ( S )-3,5-dihydroxyphenylglycine (DHPG) (100 μM) caused the dissociation between FMRP and DGL-α mRNA ( Fig. 1e ), as previously shown for other FMRP-regulated messages [22] . 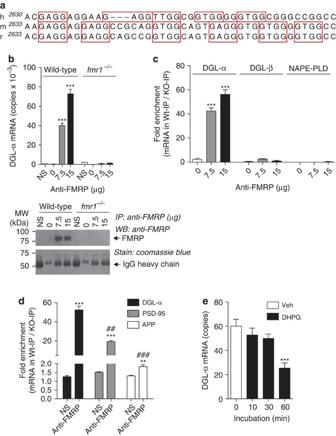Figure 1: DGL-α mRNA binds to FMRP. (a) Alignment of the coding region in human (h), mouse (m) and rat (r). DGL-α mRNAs reveal a putative G-quartet sequence within a G-rich region containing several DWGG repeats. The canonical G-quartet motif is DWGG-N(0–5)-DWGG-N(0–3)-DWGG-N(0–2)-DWGG, where D is any nucleotide except C, and W is A or U. The DWGG repeats are boxed in red. (b) Co-immunoprecipitation of FMRP with DGL-α mRNA. Brains from wild-type orfmr1−/−mice were homogenized and centrifuged at 70,000gfor 30 min. The supernatant (1 mg protein) was incubated with the indicated amounts of anti-FMRP antibody or normal serum (NS), and the immunocomplex was precipitated using protein G-sepharose beads. Top, levels of DGL-α mRNA in the immunoprecipitates were quantified by real-time quantitative PCR (n=3, ***P<0.001). Bottom, a portion of the immunoprecipitate was subjected to SDS–PAGE and western blot analyses to confirm the presence of FMRP. (c,d) Analyses of mRNAs encoding for DGL-α, DGL-β and NAPE-PLD (c) or positive control PSD-95 and amyloid precursor protein (d) in anti-FMRP-immunoprecipitates (n=3, **P<0.01 and ***P<0.001 compared with NS,##P<0.01 and###P<0.001 compared with DGL-α-anti-FMRP). Similar results were obtained usingfmr1−/−mice bred on either a FVB.129 background (b,c) or a C57BL/6J background (d). (e) DHPG-induced dissociation of DGL-α mRNA from FMRP in cultured cortical neurons. Rat primary neurons were prepared from embryonic day 18 cortex, as described55. Cells were treated with DHPG (100 μM) in culture medium and harvested at the indicated time. Levels of FMRP-bound DGL-α mRNA were determined by anti-FMRP immunoprecipitation and quantitative PCR, as described in Methods (n=5, ***P<0.001). Results are representative of at least two independent experiments. Significance was determined using two-tailed Student'st-test. Error bars represent s.e.m. Figure 1: DGL-α mRNA binds to FMRP. ( a ) Alignment of the coding region in human (h), mouse (m) and rat (r). DGL-α mRNAs reveal a putative G-quartet sequence within a G-rich region containing several DWGG repeats. The canonical G-quartet motif is DWGG-N (0–5) -DWGG-N (0–3) -DWGG-N (0–2) -DWGG, where D is any nucleotide except C, and W is A or U. The DWGG repeats are boxed in red. ( b ) Co-immunoprecipitation of FMRP with DGL-α mRNA. Brains from wild-type or fmr1 −/− mice were homogenized and centrifuged at 70,000 g for 30 min. The supernatant (1 mg protein) was incubated with the indicated amounts of anti-FMRP antibody or normal serum (NS), and the immunocomplex was precipitated using protein G-sepharose beads. Top, levels of DGL-α mRNA in the immunoprecipitates were quantified by real-time quantitative PCR ( n =3, *** P <0.001). Bottom, a portion of the immunoprecipitate was subjected to SDS–PAGE and western blot analyses to confirm the presence of FMRP. ( c , d ) Analyses of mRNAs encoding for DGL-α, DGL-β and NAPE-PLD ( c ) or positive control PSD-95 and amyloid precursor protein ( d ) in anti-FMRP-immunoprecipitates ( n =3, ** P <0.01 and *** P <0.001 compared with NS, ## P <0.01 and ### P <0.001 compared with DGL-α-anti-FMRP). Similar results were obtained using fmr1 −/− mice bred on either a FVB.129 background ( b , c ) or a C57BL/6J background ( d ). ( e ) DHPG-induced dissociation of DGL-α mRNA from FMRP in cultured cortical neurons. Rat primary neurons were prepared from embryonic day 18 cortex, as described [55] . Cells were treated with DHPG (100 μM) in culture medium and harvested at the indicated time. Levels of FMRP-bound DGL-α mRNA were determined by anti-FMRP immunoprecipitation and quantitative PCR, as described in Methods ( n =5, *** P <0.001). Results are representative of at least two independent experiments. Significance was determined using two-tailed Student's t -test. Error bars represent s.e.m. Full size image To examine whether FMRP deletion influences mGlu 5 -dependent 2-AG signalling, we used mouse brain synaptoneurosomes, a subcellular preparation enriched in resealed postsynaptic spines attached to their corresponding axon terminals [23] . As expected for previous results [10] , [11] , incubation of wild-type synaptoneurosomes with DHPG resulted in a rapid increase in DGL activity, which was dependent on both incubation time and DHPG concentration ( Fig. 2a,b ), and was accompanied by an elevation in 2-AG levels ( Fig. 2c ). These effects were not associated with changes in DGL-α content ( Fig. 2d ) and were not prevented by the translation inhibitor cycloheximide ( Supplementary Fig. S1A ), indicating that they did not require the synthesis of new DGL-α protein. In synaptoneurosomes prepared from fmr1 −/− mice, DHPG failed to stimulate DGL activity and 2-AG production ( Fig. 2a–c ), even though baseline levels of 2-AG were similar to those measured in wild-type controls ( Supplementary Fig. S1B ). The results suggest that genetic loss of FMRP disrupts mGlu 5 -dependent 2-AG signalling at excitatory synapses. 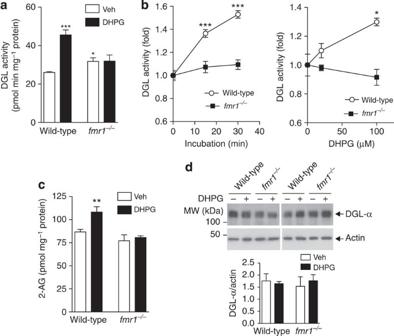Figure 2: mGlu5receptor-stimulated DGL activity and 2-AG release is disrupted infmr1−/−mice. (a) Synaptoneurosome (SN) fractions prepared from wild-type orfmr1−/−mice (1 mg ml−1) were incubated at 37 °C for 30 min in the presence of 100 μM DHPG, and DGL activity was measuredin vitrousing 10 μM diheptadecanoylglycerol as a substrate (n=4). (b) DGL activity was measured in SN fractions after incubation with various concentrations of DHPG (n=3). (c) 2-AG levels in SN fractions were measured after 45-min incubation with DHPG (100 μM) or vehicle (Veh, PBS) (n=5–9). (d). After treatment of synaptoneurosomes with DHPG, as described above, levels of DGL-α protein were measured by western blot. Representative images for DGL-α and loading control actin are shown (n=6 each). Experiments were conducted onfmr1−/−mice on C57BL/6J (a,d) or FVB.129 background (b,c). Results are representative of at least two independent experiments. Significance was determined using two-tailed Student'st-test. *P<0.05, **P<0.01 and ***P<0.001. Error bars represent s.e.m. Figure 2: mGlu 5 receptor-stimulated DGL activity and 2-AG release is disrupted in fmr1 −/− mice. ( a ) Synaptoneurosome (SN) fractions prepared from wild-type or fmr1 −/− mice (1 mg ml −1 ) were incubated at 37 °C for 30 min in the presence of 100 μM DHPG, and DGL activity was measured in vitro using 10 μM diheptadecanoylglycerol as a substrate ( n =4). ( b ) DGL activity was measured in SN fractions after incubation with various concentrations of DHPG ( n =3). ( c ) 2-AG levels in SN fractions were measured after 45-min incubation with DHPG (100 μM) or vehicle (Veh, PBS) ( n =5–9). ( d ). After treatment of synaptoneurosomes with DHPG, as described above, levels of DGL-α protein were measured by western blot. Representative images for DGL-α and loading control actin are shown ( n =6 each). Experiments were conducted on fmr1 −/− mice on C57BL/6J ( a , d ) or FVB.129 background ( b , c ). Results are representative of at least two independent experiments. Significance was determined using two-tailed Student's t -test. * P <0.05, ** P <0.01 and *** P <0.001. Error bars represent s.e.m. Full size image FMRP targets DGL-α to the perisynapse One mechanism through which FMRP deletion might affect receptor-operated 2-AG production is by altering the structure of the supramolecular complex that couples mGlu 5 receptors to DGL-α (which we refer to here as 'eCB signalosome'). To test this possibility, we immunostained for mGlu 5 or DGL-α brain sections from wild-type and fmr1 −/− mice. We first focused on the core of the ventral striatum, a brain region in which the eCB system mediates excitatory LTD [8] . Immunoperoxidase labelling for mGlu 5 or DGL-α revealed a dense punctuate distribution throughout the neuropil, which appeared to be similar between wild-type and fmr1 −/− mice ( Fig. 3a,b,g,h ). Further analyses by immunogold electron microscopy revealed a widespread presence of mGlu 5 and DGL-α in postsynaptic profiles—predominantly in dendritic spine heads that received asymmetric, putatively glutamatergic inputs from DGL-α or mGlu 5 -immunonegative axon terminals ( Fig. 3c,d,i,j ). To assess whether FMRP deletion alters the subcellular distribution of mGlu 5 and DGL-α, in three separate experiments we measured the distance along the plasma membrane between the gold particles attached to DGL-α or mGlu 5 and the closest edge of the postsynaptic density. There was no statistically detectable difference in the subcellular distribution of mGlu 5 between wild-type and fmr1 −/− mice ( n =294 and 285 synapses for wild-type and fmr1 −/− mice, respectively; Kolmogorov–Smirnov test, P =0.917) ( Fig. 3k ). By contrast, the cumulative distribution functions of the subcellular localization of DGL-α were significantly different between the two genotypes ( n =259 and 185 synapses for wild-type and fmr1 −/− mice, respectively; P =0.001) ( Fig. 3e ). This suggests that FMRP deletion selectively impairs the subcellular targeting of DGL-α in postsynaptic spine heads, without affecting the targeting of mGlu 5 . 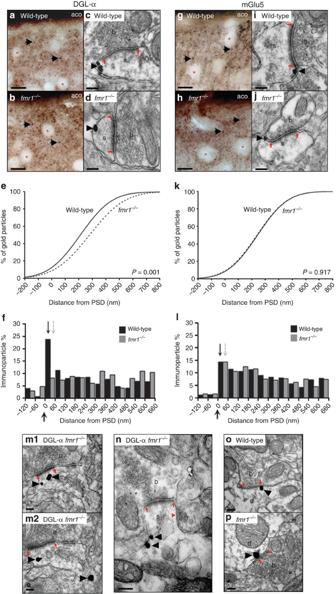Figure 3: Impaired targeting of DGL-α to the perisynaptic domain of excitatory synapses infmr1−/−mice. DGL-α immunoperoxidase labelling in wild-type (a) andfmr1−/−mice (b) reveals a similar granular staining pattern in the neuropil of the accumbens/ventral striatum (arrowheads). Medium spiny neuron somata are devoid of labelling (asterisks). aco, anterior commissure. Electron micrographs of asymmetric synapses reveal that DGL-α-positive gold particles (arrowheads) are predominantly found perisynaptically, close to the PSD (red arrows) in wild-type animals (c), but not infmr1−/−synapses (d) s, spine head; b, bouton. (e) Cumulative distribution plot of DGL-α localization in wild-type (solid line,n=259) andfmr1−/−spines (dashed line,n=185). (f) Histogram summarizing the normalized distribution of DGL-α-immunogold on the spine head membrane of wild-type mice (black arrow and black bars,n=259) andfmr1−/−mice (grey arrow and grey bars,n=185). Large arrow = edge of PSD. mGlu5immunoperoxidase labelling in wild-type (g) andfmr1−/−animals (h) depicts a similar granular labelling pattern (arrowheads) as DGL-α. Electron micrographs of asymmetric synapses containing mGlu5-immunogold labelling (arrowhead) revealed that mGlu5was predominantly found perisynaptically (red arrows) in both wild-type (i) andfmr1−/−spines (j). (k) Cumulative distribution plot of mGlu5-immunogold localization in wild-type (solid line,n=294) andfmr1−/−mice (dashed line,n=285). (l) Histogram representing the normalized distribution of mGlu5-immunogold on spine heads of wild-type (black arrow and black bars,n=294) andfmr1−/−spines (grey arrow and grey bars,n=285). The number of DGL-α-positive spines was higher infmr1−/−mice; however, the density of spine head membrane labelling was the same in both strains. Instead, a significantly higher density of DGL-α labelling was found within the spine head and neck cytoplasm (arrowheads;m1–m2) and along the spine neck membrane (black arrowheads;n). Symmetrical synapses are considered inhibitory GABAergic inputs and frequently synapse onto spine necks (red arrowhead;n) and dendritic shafts Importantly, the number of DGL-α positive symmetrical synapses were similar in wild-type (o) andfmr1−/−mice (p). Scale bars: 15 μm ina,b,gandhand 100 nm inc,d,i,j,m–p. Figure 3: Impaired targeting of DGL-α to the perisynaptic domain of excitatory synapses in fmr1 −/− mice. DGL-α immunoperoxidase labelling in wild-type ( a ) and fmr1 −/− mice ( b ) reveals a similar granular staining pattern in the neuropil of the accumbens/ventral striatum (arrowheads). Medium spiny neuron somata are devoid of labelling (asterisks). aco, anterior commissure. Electron micrographs of asymmetric synapses reveal that DGL-α-positive gold particles (arrowheads) are predominantly found perisynaptically, close to the PSD (red arrows) in wild-type animals ( c ), but not in fmr1 −/− synapses ( d ) s, spine head; b, bouton. ( e ) Cumulative distribution plot of DGL-α localization in wild-type (solid line, n =259) and fmr1 −/− spines (dashed line, n =185). ( f ) Histogram summarizing the normalized distribution of DGL-α-immunogold on the spine head membrane of wild-type mice (black arrow and black bars, n =259) and fmr1 −/− mice (grey arrow and grey bars, n =185). Large arrow = edge of PSD. mGlu 5 immunoperoxidase labelling in wild-type ( g ) and fmr1 −/− animals ( h ) depicts a similar granular labelling pattern (arrowheads) as DGL-α. Electron micrographs of asymmetric synapses containing mGlu 5 -immunogold labelling (arrowhead) revealed that mGlu 5 was predominantly found perisynaptically (red arrows) in both wild-type ( i ) and fmr1 −/− spines ( j ). ( k ) Cumulative distribution plot of mGlu 5 -immunogold localization in wild-type (solid line, n =294) and fmr1 −/− mice (dashed line, n =285). ( l ) Histogram representing the normalized distribution of mGlu 5 -immunogold on spine heads of wild-type (black arrow and black bars, n =294) and fmr1 −/− spines (grey arrow and grey bars, n =285). The number of DGL-α-positive spines was higher in fmr1 −/− mice; however, the density of spine head membrane labelling was the same in both strains. Instead, a significantly higher density of DGL-α labelling was found within the spine head and neck cytoplasm (arrowheads; m1 – m2 ) and along the spine neck membrane (black arrowheads; n ). Symmetrical synapses are considered inhibitory GABAergic inputs and frequently synapse onto spine necks (red arrowhead; n ) and dendritic shafts Importantly, the number of DGL-α positive symmetrical synapses were similar in wild-type ( o ) and fmr1 −/− mice ( p ). Scale bars: 15 μm in a , b , g and h and 100 nm in c , d , i , j , m – p . Full size image To investigate this phenomenon further, we divided the spine-head plasma membrane into 60-nm bins and calculated the frequency of gold particles within each bin. As previously shown for the hippocampus [13] , particles associated with DGL-α were concentrated in the perisynaptic zone, with a gradient that decreased towards the spine neck, and were nearly absent from the intrasynaptic domain ( Fig. 3f ). This skewed distribution was clearly detectable in the ventral striatum core of wild-type mice, but was totally absent in fmr1 −/− mutants ( Fig. 3f ). Swapping all data points in the first 60-nm bin of wild-type mice to the same data set of fmr1 −/− animals and vice versa eliminated statistical significance (Kolmogorov–Smirnov test, P =0.187 and P =0.332 for wild-type to fmr1 −/− swap and fmr1 −/− to wild-type swap, respectively). As swapping data sets in other bins did not reveal differences, the disappearance of DGL-α labelling from the perisynaptic domain may underlie the difference in the cumulative distribution functions. Furthermore, the same analytical approach revealed a biased perisynaptic localization of mGlu 5 in both wild-type and fmr1 −/− mice ( Fig. 3l ). To determine whether FMRP deletion influences the subcellular targeting of DGL-α in other forebrain structures, we examined the localization of mGlu 5 and DGL-α in the CA1 subfield of the hippocampal formation, [9] , [13] , [24] , [25] . The perisynaptic localization of mGlu 5 at hippocampal excitatory synapses was identical between fmr1 −/− and wild-type mice, whereas the localization of DGL-α was markedly impaired in fmr1 −/− mutants ( Supplementary Fig. S2 ). An economical interpretation of these findings, which is consistent with our biochemical data, is that FMRP enables the correct targeting of DGL-α and its assembly with mGlu 5 into a functional eCB signalosome at excitatory synapses throughout the forebrain. FMRP is a core component of the translational machinery in dendritic polyribosomes and has been implicated in the transport and localization of mRNAs to dendrites and synapses [3] . We reasoned therefore that, in the absence of FMRP, DGL-α mRNA might be translated ectopically. Consistent with this prediction, an analysis of 300 synapses per genotype revealed an increased average density of intracellular DGL-α labelling in the ventral striatum of fmr1 −/− mice, compared with wild-type animals (0.91 (range: 0.6–1.43) gold particles per μm 2 and 3.02 (range: 2.19–3.63) gold particles per μm 2 in wild-type and fmr1 −/− animals, respectively, normalized to background levels) ( Fig. 3m ). This increase in normalized average density was also reflected in the ratio of intracellularly localized DGL-α (14% (range: 10–17%) and 36% (range: 33–46%) of all gold particles found in dendritic spine heads in wild-type and fmr1 −/− animals, respectively). In another experiment, we assessed the presence of DGL-α labelling in a second data set of 75 random intact spines per animal. We found that fmr1 −/− spines had a higher probability of DGL-α labelling than did wild-type spines (χ 2 test, P < 0.001). In which subcellular structure was DGL-α labelling concentrated? To address this question, we divided each spine into three distinct compartments: spine-head membrane, spine-neck membrane, and head and neck cytoplasm. The number of DGL-α gold particles on the spine head membrane was very similar between wild-type and fmr1 −/− mice (χ 2 test, P= 0.696). By contrast, we found a significantly higher number of DGL-α gold particles in spine neck membrane (χ 2 test, P <0.001) ( Fig. 3n ) and cytoplasm (χ 2 test, P =0.003) of fmr1 −/− mice. In agreement with previous studies [26] , [27] , we found that dendrites in fmr1 −/− mice exhibited longer spine necks than wild-type (852±19 and 1030±24 nm in wild-type and fmr1 −/− respectively; Kolmogrov–Smirnov test, P <0.001), which might account for the higher number of DGL-α gold particles observed in these animals. However, when we calculated the density of DGL-α labelling for each spine compartment, this was also significantly higher in the fmr1 −/− necks than wild-type mice (2.29 (range: 1.63–3.01) gold particles per μm 2 and 4.67 (range: 3.63–5.85) gold particles per μm 2 in wild-type and fmr1 −/− animals, respectively). By contrast, the density of DGL-α labelling in the spine-head membrane was similar between the two strains (1.26 (range: 0.43–1.89) gold particles per μm 2 and 1.42 (range: 1.06–1.86) gold particles per μm 2 in wild-type and fmr1 −/− animals, respectively), but higher intracellular labelling was observed in fmr1 −/− mice (0.4 (range: 0.2–0.8) gold particles per μm 2 and 0.91 (range: 0.78–0.92) gold particles per μm 2 in wild-type and fmr1 −/− animals, respectively). Finally, we examined whether FMRP deletion might affect DGL-α localization at GABAergic synapses, which are also dysfunctional in fmr1 −/− mice [18] , [19] . DGL-α gold particles were found at the postsynaptic plasma membrane of both wild-type ( Fig. 3o ) and fmr1 −/− mice ( Fig. 3p ), but no statistically detectable difference was noted in their distribution (χ 2 test, P =0.6, n =150). The results suggest that genetic FMRP deletion alters the normal localization of DGL-α at excitatory, but not inhibitory, synapses of the forebrain, causing this enzyme to accumulate ectopically in the neck and cytoplasm of dendritic spines. FMRP enables eCB-LTD in ventral striatum and PFC The biochemical and ultrastructural results reported above suggest that FMRP deletion reduces 2-AG-dependent LTD at excitatory synapses of the forebrain. In acutely dissected brain slices from wild-type mice, low-frequency electrical stimulations (10 min, 10 Hz) elicited robust LTD of excitatory postsynaptic currents (EPSCs, Fig. 4a , white symbols) or extracellular field potentials (fEPSP, see Fig. 5a ) in medium spiny neurons of the ventral striatum [8] . The induction of LTD was prevented by the DGL-α inhibitor tetrahydrolipstatin (10 μM) ( Fig. 4b ), as expected from previous work [9] , [28] , and was not affected by pharmacological blockade of protein synthesis ( Supplementary Fig. S3 ). Importantly, the same low-frequency stimulations that caused LTD in wild-type mice failed to do so in fmr1 −/− mutants ( Figs 4a and 5a , black symbols). Moreover, bath applications of the mixed mGlu 1 /mGlu 5 agonist, DHPG, which consistently elicited LTD in brain slices prepared from wild-type mice, were ineffective in slices obtained from fmr1 −/− mutants ( Fig. 4c ). To evaluate whether the deficits in eCB-LTD observed in fmr1 −/− mutants extended beyond the ventral striatum, we took advantage of the fact that this brain region receives major excitatory projections from the medial PFC, a structure where mGlu 5 activation also underlies 2-AG-dependent eCB-LTD at synapses of pyramidal neuron layers 2/3 and 5/6 (refs 9 , 29 ). Similar to the ventral striatum, eCB-LTD was absent in PFC slices obtained from fmr1 −/− mutants ( Fig. 4d ). Together, these results support the idea that FMRP deletion causes a widespread impairment of mGlu 5 -dependent LTD at excitatory synapses. 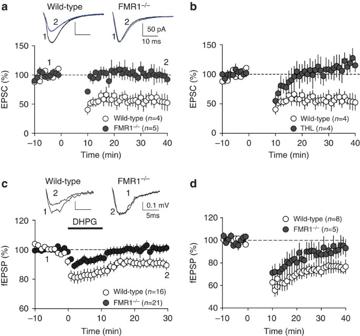Figure 4: LTD is abolished in ventral striatum and PFC offmr1−/−mice. (a) Summary graph showing whole-cell evoked EPSC amplitudes. Values are normalized to baseline before the induction of LTD and averaged per minute. Tetanic stimulation (10 min at 10 Hz starting at time 0) of PFC afferent fibres to medium spiny neurons in the ventral striatum induces a robust LTD in wild-type littermates (open symbols,n=4) but notfmr1−/−mice (filled symbols,n=5). Here as in all physiology figures,nequals the number of animals. (b) Summary graph showing averaged time courses of the experiments in which the 10 min at 10-Hz protocol was given in control ACSF (open symbols,n=4) and after pre-treatment with tetrahydrolipstatin (THL, 10 μM, filled symbols,n=4), an inhibitor of the DGL-α. Graphs show EPSC amplitudes normalized to baseline before the induction of LTD and averaged per minute. (c) Direct pharmacological activation of mGlu1/5with 50 μM (S)-DHPG induces LTD in the ventral striatum of wild-type littermates (open symbols,n=16) but notfmr1−/−mice (filled symbols,n=21). Summary graphs show excitatory postsynaptic field potentials (fEPSP) amplitudes. (d) Summary graph showing fEPSP amplitudes recorded in pyramidal neurons of the PFC. Values are normalized to baseline before the induction of LTD and averaged per minute. Tetanic stimulation (10 min at 10 Hz starting at time 0) of layers 2/3 to layers 5/6 pyramidal synapses induces a robust LTD in wild-type littermates (open symbols,n=8) but notfmr1−/−mice (filled symbols,n=5). Statistical significance was determined using Mann–WhitneyU-test. Error bars represent s.e.m. Figure 4: LTD is abolished in ventral striatum and PFC of fmr1 −/− mice. ( a ) Summary graph showing whole-cell evoked EPSC amplitudes. Values are normalized to baseline before the induction of LTD and averaged per minute. Tetanic stimulation (10 min at 10 Hz starting at time 0) of PFC afferent fibres to medium spiny neurons in the ventral striatum induces a robust LTD in wild-type littermates (open symbols, n =4) but not fmr1 −/− mice (filled symbols, n =5). Here as in all physiology figures, n equals the number of animals. ( b ) Summary graph showing averaged time courses of the experiments in which the 10 min at 10-Hz protocol was given in control ACSF (open symbols, n =4) and after pre-treatment with tetrahydrolipstatin (THL, 10 μM, filled symbols, n =4), an inhibitor of the DGL-α. Graphs show EPSC amplitudes normalized to baseline before the induction of LTD and averaged per minute. ( c ) Direct pharmacological activation of mGlu 1/5 with 50 μM ( S )-DHPG induces LTD in the ventral striatum of wild-type littermates (open symbols, n =16) but not fmr1 −/− mice (filled symbols, n =21). Summary graphs show excitatory postsynaptic field potentials (fEPSP) amplitudes. ( d ) Summary graph showing fEPSP amplitudes recorded in pyramidal neurons of the PFC. Values are normalized to baseline before the induction of LTD and averaged per minute. Tetanic stimulation (10 min at 10 Hz starting at time 0) of layers 2/3 to layers 5/6 pyramidal synapses induces a robust LTD in wild-type littermates (open symbols, n =8) but not fmr1 −/− mice (filled symbols, n =5). Statistical significance was determined using Mann–Whitney U -test. Error bars represent s.e.m. 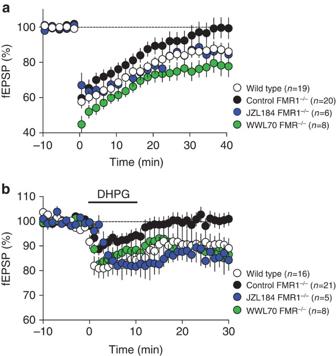Figure 5: Inhibitors of 2-AG degradation rescues eCB-dependent LTD infmr1−/−mice. (a) Normalized fEPSP amplitude infmr1−/−mice without (n=20; black symbols) or with JZL184 (1 μM; blue symbols,n=6) or WWL70 (10 μM; green symbols,n=8) pretreatment (starting 45–90 min before LTD induction) followed by the LTD induction protocol at time zero. (b) Normalized fEPSP amplitude infmr1−/−mice without (n=20; black symbols) or with JZL184 (1 μM; blue symbols,n=5) or WWL70 (10 μM; green symbols,n=8) pretreatment (starting 45–90 min before LTD induction) followed by 10-min bath perfusion with 50 μM (S)-DHPG at time zero. Statistical significance was determined using Mann–WhitneyU-test. Error bars represent s.e.m. Full size image Figure 5: Inhibitors of 2-AG degradation rescues eCB-dependent LTD in fmr1 −/− mice. ( a ) Normalized fEPSP amplitude in fmr1 −/− mice without ( n =20; black symbols) or with JZL184 (1 μM; blue symbols, n =6) or WWL70 (10 μM; green symbols, n =8) pretreatment (starting 45–90 min before LTD induction) followed by the LTD induction protocol at time zero. ( b ) Normalized fEPSP amplitude in fmr1 −/− mice without ( n =20; black symbols) or with JZL184 (1 μM; blue symbols, n =5) or WWL70 (10 μM; green symbols, n =8) pretreatment (starting 45–90 min before LTD induction) followed by 10-min bath perfusion with 50 μM ( S )-DHPG at time zero. Statistical significance was determined using Mann–Whitney U -test. Error bars represent s.e.m. Full size image To test the alternative possibility that the LTD deficit observed in fmr1 −/− mice might result from impaired CB 1 receptor function, we assessed the ability of the cannabinoid agonist CP55940 (0.01–10 μM) to inhibit synaptic transmission in slices of ventral striatum prepared from wild-type or fmr1 −/− mice. The drug's potency and efficacy were identical in the two strains ( Supplementary Fig. S4A ), indicating that CB 1 receptors function normally in fmr1 −/− mice. Moreover, tonic eCB signalling did not appear to be affected by FMRP deletion, because the selective CB 1 inverse agonist AM251 (4 μM, applied 30 min before testing) did not alter baseline excitatory transmission in the ventral striatum of wild-type or fmr1 −/− mice ( Supplementary Fig. S4B ). Thus, the lack of eCB-dependent plasticity observed in fmr1 −/− mice cannot be accounted for by alterations in CB 1 function or tonic eCB activity. We also compared the intrinsic properties of ventral striatum medium spiny neurons in wild-type and fmr1 −/− mice, and found no difference in medium spiny neurons excitability ( Supplementary Fig. S5 ). Deletion of FMRP may negatively impact the basic properties of ventral striatum excitatory synapses and, to test for this possibility, we recorded AMPA receptor-mediated spontaneous EPSCs (sEPSCs) in medium spiny neurons of both genotypes. The amplitude and frequency of AMPAR sEPSCs were similar in wild-type and fmr1 −/− mice ( Supplementary Fig. S6 ). The results rule out the possibility that modifications of excitability or basal synaptic properties of ventral striatum medium spiny neurons may be responsible for impaired eCB-LTD in fmr1 −/− mice. To test whether FMRP might influence intracellular signal transduction pathways mediating other forms of LTD, we also analysed the LTD evoked by presynaptic mGlu 2/3 receptors, which utilizes the same transduction mechanisms that are engaged by presynaptic CB 1 receptors [30] , [31] . Bath application of the selective mGlu 2/3 agonist LY379268 (100 nM) produced comparable levels of LTD in wild-type and fmr1 −/− mice ( Supplementary Fig. S7 ). Together, our experiments support the conclusion that FMRP enables mGlu 5 to initiate retrograde 2-AG signalling and elicit LTD at excitatory synapses of the forebrain. Enhancement of 2-AG signalling normalizes LTD in fmr1 −/− mice The results reported above suggest that, in fmr1 −/− mice, the failure of DGL-α to associate with mGlu 5 into a functional eCB signalosome results in a loss of eCB-LTD. We have previously shown that pharmacological blockade of intracellular 2-AG hydrolysis, which is predominantly catalysed by presynaptic MGL [16] , [32] , lowers the threshold for LTD induction at excitatory synapses of the ventral striatum [9] , [29] . We hypothesized therefore that inhibitors of 2-AG degradation might normalize LTD in fmr1 −/− mice by reinforcing 2-AG activity at residual intact synapses or, possibly, extending the reach of ectopically produced 2-AG. To test this possibility, we blocked 2-AG hydrolysis in slices using the potent and irreversible MGL inhibitor, JZL184 [33] . Brain slices were incubated with JZL184 (1 μM) for 45–90 min before LTD induction. This treatment was sufficient to restore both synaptic and pharmacologically induced LTD in slices prepared from fmr1 −/− mutants ( Fig. 5a,b ), but had no effect in slices from wild-type controls ( Supplementary Fig. S8 ). In addition, inhibition of the postsynaptic 2-AG-hydrolysing enzyme ABHD6 [29] with WWL70 (10 μM, 45–90-min incubation) also restored LTD in slices from ventral striatum of fmr1 −/− mice ( Fig. 5a,b ). The effects of JZL184 and WWL70 indicate that pharmacological blockade of either presynaptic or postsynaptic 2-AG degradation rescues eCB-dependent LTD in fmr1 −/− mice. Enhancing 2-AG corrects behavioural changes in fmr1 −/− mice When bred on a C57BL/6 background, fmr1 −/− mice display a behavioural phenotype that is characterized by elevated motor activity in an open field ( Fig. 6a,b ) and decreased aversion to the open arms of an elevated plus maze [34] ( Fig. 6c,d ). The MGL inhibitor JZL184 (16 mg kg −1 , intraperitoneal) increased brain 2-AG levels ( Supplementary Fig. S9A ) and corrected these behavioural abnormalities within 6 h of administration ( Fig. 6a–d ). In fmr1 −/− mice, JZL184 reduced the number of squares crossed ( Fig. 6a ) and the total distance travelled ( Fig. 6b ) in the open field test. The compound also reduced the number of entries and the time spent in the open arm in the elevated plus maze test ( Fig. 6c,d and Supplementary Fig. S9C, D ). By contrast, JZL184 did not significantly affect open field or elevated plus maze behaviours in wild-type mice ( Fig. 6a–d and Supplementary Fig. S9B–D ). These experiments suggest that pharmacological enhancement of 2-AG signalling normalizes two key behavioural changes observed in fmr1 −/− mice. 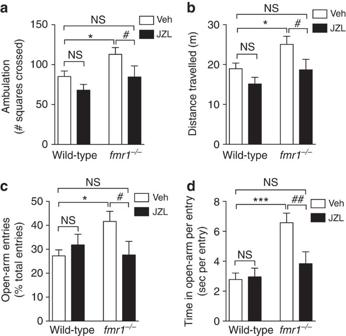Figure 6: MGL inhibition normalizes behavioural alterations infmr1−/−mice. Effects of the MGL inhibitor JZL184 on open field (a,b) and elevated plus maze (c,d) behaviours. Wild-type andfmr1−/−mice received JZL184 (JZL, 16 mg kg−1, intraperitoneal) or vehicle (Veh), and were tested 6 h after injections. Activity in the open field was measured by counting the number of squares crossed (a) and total distance travelled (b). In the elevated plus maze test, we measured percentage of open arm entries (c) and average time in open per each entry (d). Significance was determined using two-way analysis of variance withpost-hocStudent–Newman–Keuls test. NS, not significant; *P<0.05, and ***P<0.001 compared with wild-type-Veh;#P<0.05, and##P<0.01 compared withfmr1−/−-Veh (n=11 per each group). Error bars represent s.e.m. Figure 6: MGL inhibition normalizes behavioural alterations in fmr1 −/− mice. Effects of the MGL inhibitor JZL184 on open field ( a , b ) and elevated plus maze ( c , d ) behaviours. Wild-type and fmr1 −/− mice received JZL184 (JZL, 16 mg kg −1 , intraperitoneal) or vehicle (Veh), and were tested 6 h after injections. Activity in the open field was measured by counting the number of squares crossed ( a ) and total distance travelled ( b ). In the elevated plus maze test, we measured percentage of open arm entries ( c ) and average time in open per each entry ( d ). Significance was determined using two-way analysis of variance with post-hoc Student–Newman–Keuls test. NS, not significant; * P <0.05, and *** P <0.001 compared with wild-type-Veh; # P <0.05, and ## P <0.01 compared with fmr1 −/− -Veh ( n =11 per each group). Error bars represent s.e.m. Full size image In the present study, we provide three lines of evidence indicating that FMRP exerts a tight regulatory control over 2-AG-dependent retrograde signalling at excitatory synapses of the mouse forebrain. First, we show that an FMRP antibody selectively immunoprecipitates DGL-α mRNA in forebrain synaptoneurosome extracts. This is suggestive of a direct association between the two molecules, possibly through an interaction of FMRP with the G-quartet motif of DGL-α mRNA [35] . Second, we report that the normal perisynaptic colocalization of DGL-α and mGlu 5 is severely impaired in fmr1 −/− mice, indicating that FMRP is necessary for the correct targeting of DGL-α to dendritic spines. Finally, we find that FMRP deletion disrupts both mGlu 5 -stimulated 2-AG production in synaptoneurosomes and LTD at excitatory synapses of the ventral striatum and PFC. These findings suggest that FMRP may direct the assembling of DGL-α and mGlu 5 into a functional signalosome, and is essential for retrograde 2-AG transmission at glutamatergic synapses ( Fig. 7 ). Underscoring the functional significance of these results, we show that pharmacological blockade of 2-AG degradation reinstates eCB-dependent LTD and corrects key behavioural changes in fmr1 −/− mice. 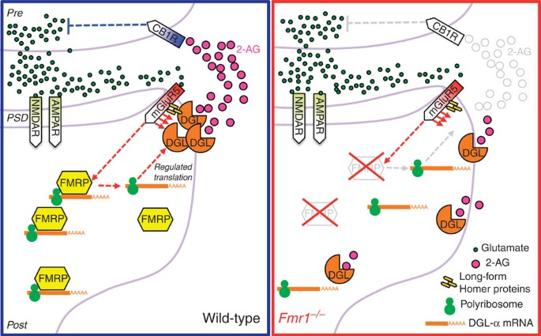Figure 7: Hypothetical role of FMRP in eCB-mediated retrograde transmission. At glutamatergic synapses of wild-type mice (left), mGlu5receptors and DGL-α are linked together in a postsynaptic signalling complex (eCB signalosome), which includes the scaffolding protein Homer. Stimulation of mGlu5receptors (mGluR5) by glutamate (green circles) increases DGL-α activity (red arrows), causing a localized rise in 2-AG levels at the perisynapse. 2-AG (red circles) travels across the synaptic cleft and inhibits glutamate release by stimulating CB1receptors (CB1R) on nerve endings. We hypothesize that FMRP helps target DGL-α to the eCB signalosome, possibly by positioning the DGL-α or Homer message(s) in specific subcellular nanodomain(s). Infmr1−/−mice (right), the lack of FMRP expression leads to disruption of this spatial organization, loss of localized 2-AG production and, consequently, impaired retrograde 2-AG-mediated signalling. AMPAR, AMPA receptors; NMDAR, NMDA receptors; PSD, postsynaptic density. Red arrows indicate intracellular signalling pathways triggered by the activation of mGlu5receptors. Molecular pathways that are impaired infmr1−/−mice are shown in grey. Figure 7: Hypothetical role of FMRP in eCB-mediated retrograde transmission. At glutamatergic synapses of wild-type mice ( left ), mGlu 5 receptors and DGL-α are linked together in a postsynaptic signalling complex (eCB signalosome), which includes the scaffolding protein Homer. Stimulation of mGlu 5 receptors (mGluR5) by glutamate (green circles) increases DGL-α activity (red arrows), causing a localized rise in 2-AG levels at the perisynapse. 2-AG (red circles) travels across the synaptic cleft and inhibits glutamate release by stimulating CB 1 receptors (CB1R) on nerve endings. We hypothesize that FMRP helps target DGL-α to the eCB signalosome, possibly by positioning the DGL-α or Homer message(s) in specific subcellular nanodomain(s). In fmr1 −/− mice ( right ), the lack of FMRP expression leads to disruption of this spatial organization, loss of localized 2-AG production and, consequently, impaired retrograde 2-AG-mediated signalling. AMPAR, AMPA receptors; NMDAR, NMDA receptors; PSD, postsynaptic density. Red arrows indicate intracellular signalling pathways triggered by the activation of mGlu 5 receptors. Molecular pathways that are impaired in fmr1 −/− mice are shown in grey. Full size image The eCB 2-AG is considered to be a primary effector of mGlu 5 -dependent plasticity in the brain [9] , [12] , [28] , but the dynamics of 2-AG signalling at central synapses are still unclear. One important question pertains to the mechanism through which mGlu 5 activation stimulates production of the 2-AG pool responsible for retrograde eCB transmission. Based on the present results, we hypothesize that the stable association of mGlu 5 and DGL-α into a multiprotein complex at the perisynaptic annulus of the dendritic spine provides a structural scaffold that allows for the localized formation of a signalling-competent pool of 2-AG, which may be distinct from the intracellular 2-AG pools involved in phospholipid remodelling and eicosanoid biosynthesis [36] , [37] . We propose to call this complex 'eCB signalosome', to signify its pivotal role in eCB-mediated retrograde transmission ( Fig. 7 ). How does the lack of FMRP expression alter the structure of the eCB signalosome? The available data suggest two possibilities. The first is that, in the absence of FMRP, the DGL-α message may be incorrectly targeted within the dendritic spines, leading to errors in the timing of DGL-α translation or the localization of the translated protein. An error in spatial mRNA delivery caused by FMRP deletion was recently demonstrated for another key postsynaptic protein, calmodulin-activated protein kinase II [38] . A second possibility is that FMRP deletion may produce an alteration in the function of Homer proteins. These scaffolding proteins bind both mGlu 5 and DGL-α [10] , and single-point mutations in the Homer-2-binding region of DGL-α result in an enzyme that retains functional activity, but is found in intracellular membrane compartments rather than the plasma membrane [10] . Notably, uncoupling of mGlu 5 from the postsynaptic Homer scaffold results in the absence of mGlu-activated retrograde 2-AG signalling at excitatory synapses [39] . Previous studies suggest a similar functional uncoupling between mGlu 5 and Homer-2 in fmr1 −/− mice, despite comparable protein levels in synaptoneurosome preparations [40] . In support of this idea, an altered balance in mGlu 5 scaffolding between short-form Homer 1a and long-form Homer proteins was found in fmr1 −/− mice [41] . The hypotheses outlined above will be tested in future experiments. The mGlu receptor theory of FRAX is based on the seminal observation that fmr1 −/− mice display a marked enhancement of a form of hippocampal LTD that depends on mGlu receptor-mediated protein synthesis [3] , [5] , [6] , [7] . Consistent with this theory, the eCB-mediated LTD induced at CA1 GABAergic synapses by pharmacological activation of mGlu 5 is similarly enhanced in fmr1 −/− mice [18] . Likewise, in the dorsal striatum of these mutants mGlu 5 -mediated eCB activity at GABAergic synapses is increased [19] . The present results, showing that eCB-LTD is abolished in the PFC and ventral striatum of fmr1 −/− mice, are only apparently in opposition with those data. Indeed, the notion that different neuron and synapse types adapt differently to the lack of FMRP is supported by a recent study showing that mGlu receptor-dependent LTP is reduced in the lateral amygdala of fmr1 −/− mice [42] . Although we found no changes in DGL-α density at GABAergic synapses, 2-AG signalling was suggested to be heterosynaptic between glutamatergic and GABAergic synapses [43] (that is, 2-AG released from dendritic spines might activate CB 1 receptors on more distant GABAergic terminals). Thus, it is possible that the shifted DGL-α localization gradient from the perisynaptic annulus to the spine neck compartment, where GABAergic synapses are often present (for example see red arrowhead in Fig. 3n ), may underlie the opposite alterations in CB 1 -dependent regulation of synaptic plasticity between these synapses (refs 18 , 19 and present study). Our findings are in line, therefore, with the core prediction of the mGlu receptor theory—namely, the idea that loss of FMRP alters most consequences of mGlu 5 activation [44] . On the other hand, the present results reveal molecular disparities between excitatory and inhibitory synapses of the same brain region, and highlight that distinct forms of LTD may also behave differentially in FRAX. While protein synthesis-dependent LTD is enhanced, presynaptic mGlu 2/3 -dependent LTD is unaffected, and finally the protein synthesis-independent, but eCB-mediated, LTD is absent. This palette of synaptic changes might underlie the complex neurobehavioural abnormalities observed in FRAX patients. Pharmacological or genetic modulation of mGlu 5 signalling normalizes various functional and structural aberrations occurring in fmr1 −/− mice—including hippocampal LTD, immature dendritic arbourization and behavioural deficits [44] . However, this approach is unlikely to restore LTD at synapses of the ventral striatum and the PFC, where we find mGlu 5 -dependent eCB production to be downregulated. We reasoned therefore that one possible alternative could be to restore eCB-mediated plasticity by reducing the degradation of its main effector, 2-AG. We used JZL184, an irreversible inhibitor of the 2-AG-degrading enzyme MGL [33] , [45] , [46] . This compound proved to be effective at restoring eCB-LTD in ventral striatum slices as well as correcting two key behavioural changes observed in fmr1 −/− mice—elevated motor activity in an open field and decreased aversion to the open arms of an elevated plus maze [34] . Despite these promising findings, the therapeutic potential of JZL184 might be limited by its ability to induce CB 1 receptor desensitization [46] . Future experimentation will be required to assess whether other classes of MGL inhibitors (for example, reversible inhibitors) [47] or agents that block additional 2-AG-hydrolysing enzymes, such as ABHD6 [29] , might normalize behaviour in fmr1 −/− mice without inducing CB 1 desensitization. Supporting the latter possibility, we observed here that acute blockade of ABHD6 re-establishes eCB-LTD in ventral striatum slices from fmr1 −/− mice. In conclusion, our results indicate that FMRP expression is necessary for the correct assembling of the eCB signalosome at glutamatergic synapses of the frontal cortex and ventral striatum core, and identify this macromolecular complex as a previously unknown substrate for FRAX, which might be targeted by therapy. Physiology Animals were treated in compliance with the European Communities Council Directive (86/609/EEC) and the United States National Institutes of Health Guide for the Care and Use of Laboratory Animals. All animals were housed, grouped and acclimated to laboratory conditions for 4 days before experiments with 12-h light/dark cycles, and access to food and water ad libitum . Male fmr1 −/− mice on a C57BL/6J genetic background [48] aged 4 to 12 weeks ( fmr1 −/− ) were used, with wild-type littermates used as control group. They were anesthetized with isoflurane and decapitated according to institutional regulations. The brain was sliced (300 μm) in the coronal plane with a vibratome (Integraslice, Campden Instruments, Loughborough, UK) in a sucrose-based solution at 4 °C (in mM: 87 NaCl, 75 sucrose, 25 glucose, 5 KCl, 21 MgCl 2 , 0.5 CaCl 2 and 1.25 NaH 2 PO 4 ). Immediately after cutting, slices were stored at room temperature in a low-calcium artificial cerebrospinal fluid (low Ca–ACSF) that contained (in mM): 130 NaCl, 11 glucose, 2.5 KCl, 2.4 MgCl 2 , 1.2 CaCl 2 , 23 NaHCO 3 and 1.2 NaH 2 PO 4 , and was equilibrated with 95% O 2 /5% CO 2 until the time of recording. Whole-cell patch-clamp of visualized medium spiny neurons, PFC pyramidal neurons and field potential recordings were made in coronal slices containing the ventral striatum or the PFC as previously described [8] , [9] , [49] , [50] . For more details, see Supplementary Methods . All values are given as mean±s.e.m. For all experiments, n corresponds to the number of animals tested for each condition. Data were analysed using Clampfit 10 (Molecular Devices, Sunnyvale, USA). Unless otherwise stated, the statistical test used was a Mann–Whitney U -test performed with GraphPad Prism (GraphPad Software, La Jolla, CA) and significance determined by P <0.05. The magnitude of LTD was calculated by comparing average responses (30–40 min) after induction to baseline-averaged responses before induction protocol (increased stimulation for 10 min at 10 Hz). Picrotoxin, THL and anisomycin were from Sigma (St Quentin Fallavier, France). 6,7-dinitroquinoxaline-2,3-dione (DNQX), (1R,3R,4R)-3-[2-hydroxy-4-(1,1-dimethylheptyl)-phenyl]-4-(3-hydroxypropyl)-cyclohexan-1-ol (CP55940), DHPG, AM251, WWL70 and JZL184 were from Tocris (Bristol, UK). Other chemicals were of the highest commercial grade available. Biochemistry Male fmr1 −/− mice (FVB.129P2-Fmr1 tm1Cgr /J) and wild-type control mice (FVB.129P2-Pde6b + Tyr c−ch /AntJ) from Jackson Laboratories (Bar Harbor, ME), aged between 6 to 10 weeks, or adult male fmr1 −/− mice on C57BL/6J background (Fmr1 KO2) were used for the biochemical studies. All procedures met the National Institutes of Health guidelines for the care and use of laboratory animals and were approved by the University of California, Irvine, Institutional Animal Care and Use Committee. All manipulations of brain homogenates were performed at 4 °C [51] . Synaptoneurosomes were prepared from whole brains of wild-type or fmr1 −/− mice. Briefly, mice were quickly decapitated, brains were removed and homogenized by 20 strokes with a glass-Teflon homogenizer in 10 ml of homogenizing buffer (118 mM NaCl, 4.7 mM KCl, 1.2 mM MgSO 4 , 2.5 mM CaCl 2 , 1.53 mM KH 2 PO 4 , 212.7 mM glucose, 1 mM DTT, pH7.4, and protease inhibitor) and filtered through a series of polypropylene filters (twice through 100 μm and once through 10 μm (BD Filcon). Filtrates were spun briefly (1,000 g , 15 min) and the pellets were reconstituted in 3 ml of homogenizing buffer at a protein concentration of 1 mg ml −1 . Dissected brain regions were homogenized in methanol (1 ml) containing [ 2 H 8 ]-2-AG and N-heptadecanoylethanolamide (Cayman Chemicals, Ann Arbor, MI, USA) as internal standards. Protein concentration was determined in the homogenate to normalize samples using the bicinchinonic acid protein assay (Pierce, Rockford, IL, USA). Lipids were extracted with chloroform (2 ml) and water (1 ml), and further fractionated by open-bed silica gel column chromatography, as previously described [52] . Lipids were reconstituted in chloroform, loaded onto small glass columns packed with Silica Gel G (60-˚ 230–400 Mesh ASTM; Whatman, Clifton, NJ, USA) and washed with 2 ml of chloroform. 2-AG were eluted with 1 ml of chloroform/methanol (9:1, vol/vol). Eluates were dried under N 2 and reconstituted in chloroform/methanol (1:3, 50 μl) for liquid chromatography/mass spectrometry (LC/MS) analyses. An 1100-LC system coupled to a 1946A-MS detector (Agilent Technologies, Inc., Palo Alto, CA, USA) equipped with an electrospray ionization interface was used to measure anandamide and 2-AG levels in lipid extracts. Lipids were separated using a XDB Eclipse C18 column (50×4.6 mm i.d., 1.8 μm, Zorbax), eluted with a gradient of methanol in water (from 75 to 85% in 2.5 min, to 90% in 7.5 min, to 100% in 14 min and to 75% in 20 min) at a flow rate of 1.0 ml min −1 . Column temperature was kept at 40 °C. MS detection was in the positive ionization mode, capillary voltage was at 3 kV and fragmentor voltage varied from 120 V. N 2 was used as drying gas at a flow rate of 13 l min −1 and temperature of 350 °C. Nebulizer pressure was set at 60 PSI. Quantifications were conducted using an isotope-dilution method [52] by monitoring Na + adducts of the molecular ions ([M+Na] + ) in the selected ion-monitoring mode. Quantification limits for 2-AG was 0.4 pmol. For reverse transcriptase-PCR and quantitative PCR and immunoprecipitation, detailed procedures are provided in Supplementary Methods . Results are expressed as the mean±s.e.m. Statistical significance was evaluated using the Student's t -test. Animal behaviour Adult male fmr1 −/− C57BL/6J mice were used for the animal behaviour studies. For open field and elevated plus maze, detailed procedures provided in Supplementary Methods [53] , [54] . Anatomy Experiments were performed according to the guidelines of the institutional ethical code and the Hungarian Act of Animal Care and Experimentation (1998; XXVIII. Section 243/1998). Adult male C57BL/6J mice (three wild-type and three fmr1 −/− mice (8 weeks old) were deeply anesthetized with a mixture of ketamine–xylazine (25 mg ml −1 ketamine, 5 mg ml −1 xylazine, 0.1% w/w pipolphen in H 2 O; 1 ml per 100 g , intraperitoneal). Animals were then perfused transcardially with 0.9% saline for 2 min, followed by 100 ml of fixative containing 4% paraformaldehyde and 0.1% glutaraldehyde in 0.1 M phosphate buffer (PB), pH 7.4, for 20 min. After perfusion, the brain was removed from the skull, cut into blocks, post-fixed for 2 h and washed in PB. The blocks containing the ventral striatum were sliced into 50-μm-thick coronal sections of the brain with a Leica VTS-1000 vibratome (Vibratome, St Louis, MO, USA). After slicing and extensive washing in 0.1 M PB, the sections were incubated in 10% sucrose for 15 min and 30% sucrose overnight, followed by freeze thawing over liquid nitrogen four times. Subsequently, all washing steps and dilutions of the antibodies were performed in 0.05 M Tris-buffered saline (TBS), pH 7.4. After extensive washing in TBS, the sections were blocked in 5% normal goat serum for 45 min and then incubated in rabbit anti-DGL-α (1:3,000, 'INT'; [13] ) or rabbit anti-mGlu 5 (1:1,000, AB5675, Millipore, Billerica, MA, USA) for a minimum of 48 h at 4 °C. In the immunoperoxidase staining procedure, after primary antibody incubations, the sections were treated with biotinylated goat anti-rabbit IgG (1:400, Vector Laboratories) for 2 h and after three washes in TBS, with avidin biotinylated–horseradish peroxidase complex (1:500; Elite ABC; Vector Laboratories) for 1.5 h. After extensive washing, the immunoperoxidase reaction was developed using 3,3′-diaminobenzidine as the chromogen. In the immunogold staining procedure, after the primary antibody incubation, the sections were washed extensively in TBS before incubation in 0.8 nm gold-conjugated goat anti-rabbit secondary antibody (1:50; AURION, Wageningen, The Netherlands), overnight at 4 °C. Then sections were silver intensified using the silver enhancement system R-GENT SE-EM according to the kit protocol (AURION). After development of both types of immunolabelling, the sections were treated with osmium tetroxide (0.5% for immunogold labelling, 1% for immunoperoxidase reaction) in 0.1M PB for 20 min (at 4 °C for immunogold labelling) and dehydrated in an ascending series of ethanol and acetonitrile, before being embedded in Durcupan (ACM, Fluka, Buchs, Switzerland). During dehydration, sections were treated with 1% uranyl acetate in 70% ethanol for 15 min (at 4 °C for immunogold labelling). Immunoperoxidase-labelled sections were imaged with a Nikon Eclipse 80i microscope (Nikon Instruments Europe B.V., Amsterdam, The Netherlands) and light micrographs were captured with a DS-Fi1 digital camera (Nikon Instruments Europe B.V., Amsterdam, The Netherlands). For electron microscopy analysis, areas of interest in the ventral striatum core were removed from Durcupan-embedded sections, then re-embedded and re-sectioned. Ultrathin (60 nm) sections were collected on Formvar-coated single-slot grids and stained with lead citrate. Electron micrographs were taken at ×40,000 magnifications with a Hitachi 7100 electron microscope (Tokyo, Japan). Quantitative analysis of the distribution of DGL -α and mGlu 5 in dendritic spines: see Supplementary Methods . How to cite this article: Jung, K.-M. et al . Uncoupling of the endocannabinoid signalling complex in a mouse model of fragile X syndrome. Nat. Commun. 3:1080 doi: 10.1038/ncomms2045 (2012).